The ubiquitin ligase HACE1 regulates Golgi membrane dynamics during the cell cycle Partitioning of the Golgi membrane into daughter cells during mammalian cell division occurs through a unique disassembly and reassembly process that is regulated by ubiquitination. However, the identity of the ubiquitin ligase is unknown. Here we show that the Homologous to the E6-AP Carboxyl Terminus (HECT) domain containing ubiquitin ligase HACE1 is targeted to the Golgi membrane through interactions with Rab proteins. The ubiquitin ligase activity of HACE1 in mitotic Golgi disassembly is required for subsequent postmitotic Golgi membrane fusion. Depletion of HACE1 using small interfering RNAs or expression of an inactive HACE1 mutant protein in cells impaired postmitotic Golgi membrane fusion. The identification of HACE1 as a Golgi-localized ubiquitin ligase provides evidence that ubiquitin has a critical role in Golgi biogenesis during the cell cycle. Mitosis requires the duplication and even partitioning of all cellular components into the daughter cells. In mammalian cells, inheritance of the Golgi apparatus during cell division occurs through a unique disassembly and reassembly process [1] , [2] . The Golgi is fragmented at the onset of mitosis to disperse the stacks, which then undergo further vesiculation. This gives thousands of vesicles that are distributed throughout the cytoplasm [3] . Studies using a cell-free assay that reconstitutes mitotic Golgi fragmentation, [4] , [5] , [6] , [7] showed that mitotic Golgi disassembly involves two processes: cisternal unstacking and membrane vesiculation. Unstacking is mediated by mitotic kinases that phosphorylate the Golgi-stacking proteins GRASP65 and GRASP55 (refs 8 , 9 , 10 , 11 ). In interphase cells, GRASP proteins form oligomers that hold the membranes in stacks. During mitosis, phosphorylation of GRASPs leads to de-oligomerization of the proteins and cisternal unstacking. Vesiculation of the unstacked cisternae occurs through continuous formation of coat protein complex I vesicles, which is mediated by the small GTPase ARF1 (ADP-ribosylation factor 1) and the coatomer complex [12] . Phosphorylation of Golgi tethering proteins, such as GM130, disrupts membrane fusion, and continuous COPI vesicle budding without fusion results in vesiculation of the Golgi membranes during mitosis [13] . During telophase, Golgi vesicles are distributed equally between daughter cells, where they are assembled into stacks and ribbons. Postmitotic Golgi reassembly is mediated by membrane fusion to form single cisternae and by cisternal stacking. Postmitotic Golgi membrane fusion is mediated by two AAA (ATPases Associated with various cellular Activities) ATPases, N -ethylmaleimide-sensitive factor (NSF) and p97 (also referred to as valosin-containing protein, or Cdc48 in yeast), which work together with their adaptor proteins [14] , [15] , [16] , [17] , [18] , [19] . Golgi membrane restacking is mediated by dephosphorylation and subsequent re-oligomerization of Golgi stacking proteins [2] , [6] , [8] , [9] , [10] , [11] , [20] . Several converging lines of evidence have suggested that monoubiquitination has an essential role in the regulation of postmitotic Golgi membrane fusion. First, monoubiquitination occurs during mitotic Golgi disassembly and is required for subsequent Golgi reassembly [20] . Second, the p97/p47 complex binds to monoubiquitin through the UBA domain of the adaptor protein p47. Inhibition of the p47-ubiquitin interaction suppresses p97-mediated Golgi membrane fusion [20] . Third, VCIP135, a cofactor of the p97/p47 complex, is a deubiquitinating enzyme whose activity is required for postmitotic Golgi reassembly [21] . Finally, proteasome activity is not involved in either Golgi disassembly or reassembly [21] . These data suggest that cycles of addition and removal of ubiquitin to and from substrates is necessary for Golgi reassembly. The role of ubiquitination in Golgi membrane fusion is likely not restricted to the p97/p47 complex, as it has been shown that another required ATPase, NSF, binds to GATE-16, a ubiquitin-like protein [22] , [23] . These results suggest that ubiquitination may operate as a general mechanism to regulate Golgi membrane dynamics during the cell cycle. Both NSF- and p97-mediated Golgi reassembly require syntaxin 5, but these two pathways contribute non-additively to cisternal regrowth [15] . This suggests that they may have distinct roles in postmitotic Golgi membrane fusion, but the coordination between the two pathways has not been elucidated. Further understanding of the underlying mechanism of ubiquitin in the regulation of Golgi membrane dynamics during cell division requires identification of the ubiquitin ligase on the Golgi membranes. Here we show that HACE1, a HECT domain (Homologous to the E6-AP Carboxyl Terminus)-containing ubiquitin ligase, is involved in this process. HACE1 is recruited to the Golgi membrane via interaction with Rab1, and regulates postmitotic Golgi membrane fusion both in vitro and in vivo . The identification of HACE1 as a Golgi-localized ubiquitin ligase provides further evidence that ubiquitin has a critical role in Golgi biogenesis during the cell cycle. Identification of HACE1 as a Rab-interacting protein Rab proteins have been shown to be important for membrane organization [24] . In an effort to identify Rab-interacting proteins using an affinity chromatography-based proteomic approach [25] , we identified HACE1, which binds specifically to the guanosine-5′-triphosphate (GTP)-bound state of Rab4 ( Fig. 1a ). The HACE1 cDNA was cloned from a human cDNA library. It consisted of 909 amino acids and migrated at 100 kDa on an SDS–PAGE gel. HACE1 contains six ankyrin repeats and a HECT domain [26] , a defining feature of one family of ubiquitin E3 ligases. Using a thioester bond formation assay containing ubiquitin, an E1-activating enzyme, the E2 conjugating enzyme UbcH7 and recombinant HACE1, we demonstrated that wild-type (WT) HACE1 is capable of catalyzing the formation of thioester bonds, but the inactive C876A (CA) mutant is not ( Fig. 1b ). This result is consistent with previous reports that HACE1 functions as an active ubiquitin ligase [26] , [27] . 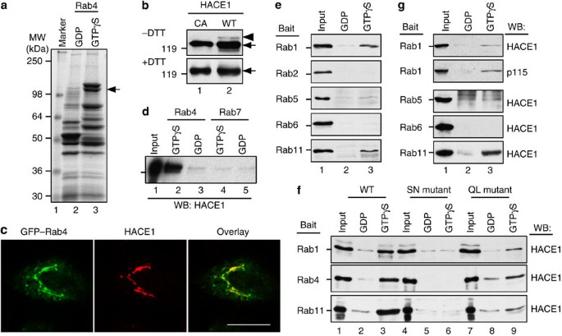Figure 1: HACE1 binds to Golgi-associated Rab proteins. (a) HACE1 binds Rab4–GTP. Immobilized GST-tagged Rab4 was incubated with bovine brain cytosol in the presence of GDP or GTPγS. After washing, the bound proteins were eluted and analysed by SDS–PAGE and coomassie blue staining. Specific bands in the GTPγS lane were excised and identified by mass spectrometry. The arrow indicates HACE1. (b) HACE1 exhibits ubiquitin ligase activityin vitro. A thioester bond formation assay was performed using the C876A (CA) point mutant and WT recombinant HACE1 protein, ubiquitin, E1-activating enzyme and the E2-conjugating enzyme UbcH7. Following incubation, the reactions were mixed with SDS buffer±DTT and boiling. HACE1 was detected by western blot. The arrows indicate HACE1 and the arrowhead indicates Ub-HACE1. Note that the Ub-HACE1 band was observed in the absence of DTT with WT HACE1. (c) HACE1 colocalizes with Rab4 in the perinuclear region. Immunofluorescence images of A431 cells expressing GFP–Rab4 (in green) and stained for HACE1 (in red). Note that HACE1 colocalizes with Rab4 in the perinuclear region, while additional Rab4 signal is found in the cytoplasm. Scale bar, 20 μm. (d) HACE1 directly binds Rab4–GTP but not Rab7. Immobilized GST-tagged Rab4 and Rab7 were incubated with purified recombinant HACE1 in the presence of GDP or GTPγS. After washing, HACE1 was detected by western blot for HACE1. Input, 5%. (e) Recombinant HACE1 binds Rab1 and 11 but not Rab2, 5 and 6. Input, 5%. (f) HACE1 interacts with Rabs in a nucleotide-dependent manner. Same as in (e) but with the WT Rab1, 4 and 11 (WT, lanes 1–3), and their 'GDP' (SN mutant, lanes 4–6) and 'GTP' (QL mutant, lanes 7–9) locked forms. Input, 5%. (g) Endogenous HACE1 binds Golgi-associated Rabs. As in (d) but using HeLa cell lysates instead of purified HACE1 protein. Input, 10%. Lines on the left of the blots in (d–g) indicate the molecular weight marker of 95 kDa. Figure 1: HACE1 binds to Golgi-associated Rab proteins. ( a ) HACE1 binds Rab4–GTP. Immobilized GST-tagged Rab4 was incubated with bovine brain cytosol in the presence of GDP or GTPγS. After washing, the bound proteins were eluted and analysed by SDS–PAGE and coomassie blue staining. Specific bands in the GTPγS lane were excised and identified by mass spectrometry. The arrow indicates HACE1. ( b ) HACE1 exhibits ubiquitin ligase activity in vitro . A thioester bond formation assay was performed using the C876A (CA) point mutant and WT recombinant HACE1 protein, ubiquitin, E1-activating enzyme and the E2-conjugating enzyme UbcH7. Following incubation, the reactions were mixed with SDS buffer±DTT and boiling. HACE1 was detected by western blot. The arrows indicate HACE1 and the arrowhead indicates Ub-HACE1. Note that the Ub-HACE1 band was observed in the absence of DTT with WT HACE1. ( c ) HACE1 colocalizes with Rab4 in the perinuclear region. Immunofluorescence images of A431 cells expressing GFP–Rab4 (in green) and stained for HACE1 (in red). Note that HACE1 colocalizes with Rab4 in the perinuclear region, while additional Rab4 signal is found in the cytoplasm. Scale bar, 20 μm. ( d ) HACE1 directly binds Rab4–GTP but not Rab7. Immobilized GST-tagged Rab4 and Rab7 were incubated with purified recombinant HACE1 in the presence of GDP or GTPγS. After washing, HACE1 was detected by western blot for HACE1. Input, 5%. ( e ) Recombinant HACE1 binds Rab1 and 11 but not Rab2, 5 and 6. Input, 5%. ( f ) HACE1 interacts with Rabs in a nucleotide-dependent manner. Same as in ( e ) but with the WT Rab1, 4 and 11 (WT, lanes 1–3), and their 'GDP' (SN mutant, lanes 4–6) and 'GTP' (QL mutant, lanes 7–9) locked forms. Input, 5%. ( g ) Endogenous HACE1 binds Golgi-associated Rabs. As in ( d ) but using HeLa cell lysates instead of purified HACE1 protein. Input, 10%. Lines on the left of the blots in ( d – g ) indicate the molecular weight marker of 95 kDa. Full size image When examined by fluorescence microscopy, both Rab4 and HACE1 were concentrated in the perinuclear region, which appeared to be the Golgi apparatus ( Fig. 1c ). In addition to the Golgi, Rab4, but not HACE1, was also found on endosomal membranes that were irregularly shaped and dispersed throughout the cytosol ( Fig. 1c ). Because HACE1 binds to Rab4, which is only partially localized to the Golgi, we examined whether HACE1 also interacts with other Rabs, including those localized on the Golgi, using a well-established Rab pull-down assay [25] , [28] . Immobilized glutathione S-transferase (GST)-tagged Rab proteins were incubated with purified recombinant HACE1 in the presence of guanosine diphosphate (GDP) or guanosine-5′- O -(3-thiotriphosphate) GTPγS, and the presence of HACE1 in the bound fraction was detected by western blot. As shown in Figure 1d, e , HACE1 bound to Rab1, Rab4 and Rab11 in a GTP-dependent manner, but not to Rab2, 5, 6 and 7, irrespective of the nucleotide used. To confirm the interaction, we tested HACE1 binding to the GDP- (Rab1S25N, Rab4S22N and Rab11S25N) and GTP-restricted (Rab1Q67L, Rab4Q67L and Rab11Q70L) mutants of Rab1, 4 and 11. As shown in Figure 1f , HACE1 bound to the WT and the active GTP forms of all three Rabs but not their inactive mutants. Using HeLa cell lysate, we further confirmed that endogenous HACE1 bound to Rab1–GTP in a similar pattern as p115, a protein known to interact with Rab1. A strong interaction was also observed for Rab11, but no interactions were detected for Rab5 or Rab6 ( Fig. 1g ). These results demonstrate that HACE1 interacts with Rab1, 4 and 11 in a GTP-dependent manner. HACE1 is associated with Golgi membranes HACE1 lacks a transmembrane domain and has been shown to be associated, at least in part, with the endoplasmic reticulum (ER) in NIH3T3 cells [26] . NIH3T3 cells are not often used in studies of Golgi proteins, partially because of their relatively small size. Considering the interactions of HACE1 with Rab1, 4 and 11, which are at least partially localized to Golgi membranes [28] , [29] , [30] , [31] , [32] , we determined whether HACE1 localizes to the Golgi during interphase in normal rat kidney (NRK) cells. A fraction of HACE1 colocalized with GRASP65, a Golgi marker, and the rest of the protein appeared to be cytosolic ( Fig. 2a ), similar to the results observed in A431 cells ( Fig. 1c ). Both the Golgi and cytosolic signals were diminished by the addition of recombinant HACE1 protein to displace the antibodies ( Fig. 2b , anti-HACE1+peptide), suggesting that the antibody had high specificity. 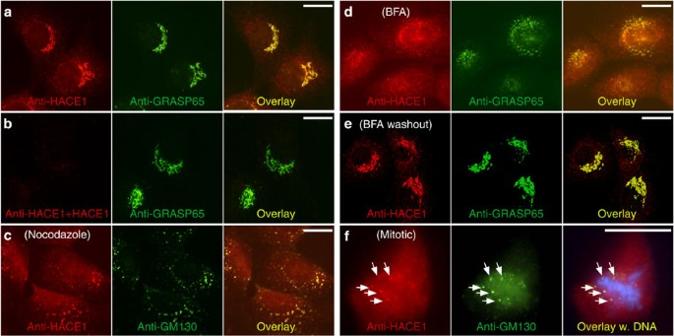Figure 2: HACE1 is concentrated on the Golgi apparatus. (a) HACE1 is concentrated on the Golgi in interphase cells. NRK cells were immunostained with an affinity-purified polyclonal antibody to HACE1 (left panel, in red) and a monoclonal antibody to GRASP65 (middle panel, in green). (b) The HACE1 antibodies are specific. Same as in (a), except the HACE1 antibodies were preincubated with purified HACE1 recombinant protein to quench the antibodies. Note that the HACE1 fluorescence was displaced by the recombinant HACE1. (c) HACE1 is associated with Golgi fragments after nocodazole treatment. NRK cells were treated with 0.5 μg ml−1nocodazole for 2 h and stained for HACE1 and GM130. (d) Brefeldin A (BFA) treatment leads to the dispersal of HACE1 in the cell. NRK cells were treated with 5 μg ml−1BFA for 2 h and analysed as in (a). (e) BFA washout. After the removal of BFA, cells were further incubated in growth media for 2 h and stained for HACE1 and GRASP65. (f) HACE1 is partially associated with the Golgi fragments in prometaphase cells. Prometaphase NRK cells stained for HACE1 (red), GM130 (green) and DNA (blue). Note that HACE1 is localized on the mitotic Golgi fragments (indicated by arrows). Scale bars in all panels, 10 μm. Figure 2: HACE1 is concentrated on the Golgi apparatus. ( a ) HACE1 is concentrated on the Golgi in interphase cells. NRK cells were immunostained with an affinity-purified polyclonal antibody to HACE1 (left panel, in red) and a monoclonal antibody to GRASP65 (middle panel, in green). ( b ) The HACE1 antibodies are specific. Same as in ( a ), except the HACE1 antibodies were preincubated with purified HACE1 recombinant protein to quench the antibodies. Note that the HACE1 fluorescence was displaced by the recombinant HACE1. ( c ) HACE1 is associated with Golgi fragments after nocodazole treatment. NRK cells were treated with 0.5 μg ml −1 nocodazole for 2 h and stained for HACE1 and GM130. ( d ) Brefeldin A (BFA) treatment leads to the dispersal of HACE1 in the cell. NRK cells were treated with 5 μg ml −1 BFA for 2 h and analysed as in ( a ). ( e ) BFA washout. After the removal of BFA, cells were further incubated in growth media for 2 h and stained for HACE1 and GRASP65. ( f ) HACE1 is partially associated with the Golgi fragments in prometaphase cells. Prometaphase NRK cells stained for HACE1 (red), GM130 (green) and DNA (blue). Note that HACE1 is localized on the mitotic Golgi fragments (indicated by arrows). Scale bars in all panels, 10 μm. Full size image We then treated the cells with chemicals known to affect the Golgi structure. Nocodazole treatment leads to fragmentation of the Golgi ribbon. After nocodazole treatment, HACE1 colocalized with the Golgi remnants indicated by GM130 ( Fig. 2c ). Brefeldin A (BFA) treatment leads to Golgi membrane fusion with the ER. In the presence of BFA, Golgi remnants, marked by GRASP65, were dispersed throughout the cell along with HACE1 ( Fig. 2d ). After BFA was washed out, HACE1 accumulated in perinuclear regions where the Golgi membranes were concentrated ( Fig. 2e ). Finally, in mitotic cells with fragmented Golgi membranes, HACE1 associated with mitotic Golgi clusters, as determined by the presence of GM130 ( Fig. 2f ). Further microscopic analysis indicated that HACE1 colocalized well with the cis -Golgi markers GRASP65 and GM130 ( Fig. 2 ), and with GFP tagged GalNac-T2 ( N -acetylgalactosaminyltransferase 2), a Golgi enzyme localized throughout the Golgi stack ( Supplementary Fig. S1 ) [33] . HACE1 also colocalized with the medial- and trans -Golgi markers α-mannosidase II [34] and syntaxin 6 (ref. 35 ), though to a less extent compared with the cis -Golgi markers. In addition, it showed partial colocalization with the ER–Golgi intermediate compartment marker ERGIC53 (ref. 36 ) in the perinuclear region where Golgi membranes were concentrated. Colocalization of HACE1 with cis -Golgi markers, compared with other Golgi compartment markers, was more evident when the Golgi apparatus was fragmented by nocodazole treatment ( Fig. 2c ; Supplementary Fig. S1 ). Biochemical analysis also confirmed the association of HACE1 with Golgi membranes. Western blot of cell lysate prepared from unsynchronized interphase NRK cells and nocodazole blocked mitotic cells detected one major band of ∼ 100 kDa ( Fig. 3a ). When subcellular membrane organelles were separated using equilibrium sucrose gradients, the distribution of HACE1 was similar to the Golgi markers GM130, GRASP65, syntaxin 5 and Gos28 but was different from the ER markers Sec61 and protein disulphide isomerase (PDI, Fig. 3b ). Taken together, these results show that HACE1 is associated with Golgi membranes. 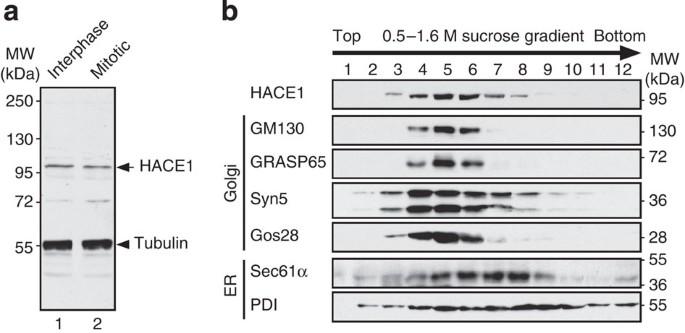Figure 3: HACE1 is a ubiquitin ligase bound to Golgi membranes. (a) The affinity-purified HACE1 antibody recognizes one major band in NRK cells. Western blot of non-synchronized interphase and nocodazole-treated mitotic NRK cell lysates for HACE1 and tubulin. (b) HACE1 colocalizes with the Golgi in sucrose gradients. Postnuclear supernatant (PNS) from interphase NRK cells was fractionated by equilibrium centrifugation on a sucrose gradient (0.5–1.6 M). Membranes from each fraction were pelleted and equal volumes were analysed by western blot for the indicated proteins. Golgi membranes were enriched in fraction 5 (with about 0.8 M sucrose), while ER membranes are more widely distributed and concentrated in heavier fractions. Figure 3: HACE1 is a ubiquitin ligase bound to Golgi membranes. ( a ) The affinity-purified HACE1 antibody recognizes one major band in NRK cells. Western blot of non-synchronized interphase and nocodazole-treated mitotic NRK cell lysates for HACE1 and tubulin. ( b ) HACE1 colocalizes with the Golgi in sucrose gradients. Postnuclear supernatant (PNS) from interphase NRK cells was fractionated by equilibrium centrifugation on a sucrose gradient (0.5–1.6 M). Membranes from each fraction were pelleted and equal volumes were analysed by western blot for the indicated proteins. Golgi membranes were enriched in fraction 5 (with about 0.8 M sucrose), while ER membranes are more widely distributed and concentrated in heavier fractions. Full size image HACE1 is targeted to the Golgi membrane by Rab1 If Rabs target HACE1 to the Golgi, inhibition of Rab activity may affect HACE1 Golgi localization. We therefore used WT and mutant Rabs to test this hypothesis. Expression of WT Rabs did not affect HACE1 Golgi localization or the Golgi structure ( Fig. 4 ; Supplementary Fig. S2 ). In addition, WT Rab1, 4 and 11, but not Rab5, were partially concentrated on Golgi membranes ( Figs 1c and 4 ; Supplementary Fig. S2 ). Expression of the active Rab1 Q67L mutant had no effect on HACE1 localization or Golgi morphology. In contrast, expression of the S25N mutant at a relatively low level ( Supplementary Fig. S2g ) disrupted HACE1 Golgi localization ( Fig. 4d ). Furthermore, expression of the Rab1 S25N mutant also caused Golgi fragmentation ( Fig. 4h ), which is consistent with previous reports [37] , and suggests that HACE1 may serve as a Rab1 effector required for Golgi integrity. Expression of Rab4, 11 and their mutants had no effect on HACE1 Golgi localization or the Golgi organization ( Fig. 4 ; Supplementary Fig. S2 ). Taken together, our data suggest that the interaction of HACE1 with Rab1 is important for HACE1 Golgi localization and function. 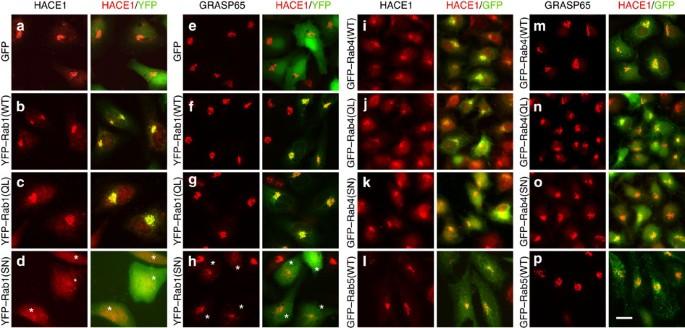Figure 4: Expression of an inactive Rab1 mutant interrupts HACE1 localization and Golgi structure. HeLa cells expressing GFP (a,e), YFP–Rab1 WT or mutant constructs (b–d,f–h), GFP–Rab4 WT or mutant constructs (i–k,m–o) or GFP–Rab5 (l,p) as indicated were immunostained for HACE1 (a–dandi–l) or GRASP65 (e–handm–p), which are shown on the left in red. The overlays with the YFP or GFP signals (in green) are shown on the right. Asterisks indicate cells expressing the Rab1 (SN) mutant, which have HACE1 dispersed from the Golgi membranes (d) and fragmented Golgi (h). Scale bars in all panels, 20 μm. Figure 4: Expression of an inactive Rab1 mutant interrupts HACE1 localization and Golgi structure. HeLa cells expressing GFP ( a , e ), YFP–Rab1 WT or mutant constructs ( b – d , f – h ), GFP–Rab4 WT or mutant constructs ( i – k , m – o ) or GFP–Rab5 ( l , p ) as indicated were immunostained for HACE1 ( a – d and i – l ) or GRASP65 ( e – h and m – p ), which are shown on the left in red. The overlays with the YFP or GFP signals (in green) are shown on the right. Asterisks indicate cells expressing the Rab1 (SN) mutant, which have HACE1 dispersed from the Golgi membranes ( d ) and fragmented Golgi ( h ). Scale bars in all panels, 20 μm. Full size image HACE1 is required for postmitotic Golgi membrane fusion To test the role of HACE1 in the formation of Golgi structure, we expressed myc-tagged WT and mutant HACE1 in HeLa cells and examined Golgi morphology. Deletion of the HECT domain (amino acids 1–553 lacking the HECT domain, designated HACE1 ΔC) or mutation of cysteine 876 to analine (the CA mutant, Fig. 5a ) abolished the ubiquitin ligase activity [27] . The exogenously expressed proteins were partially localized on the Golgi examined by fluorescence microscopy ( Fig. 5b ). Expression of the WT HACE1 did not affect the integrity of the Golgi structure. However, expression of the CA or the ΔC mutant led to Golgi fragmentation; with 33.4±1.4 and 49.8±0.1% of the cells had fragmented Golgi, respectively, which was significantly higher than cells transfected with WT HACE1 (9.6±1.0%) or with the vector alone (8.9±0.1%; Fig. 5 ). These results suggest that HACE1 ubiquitin ligase activity is involved in maintaining Golgi integrity. 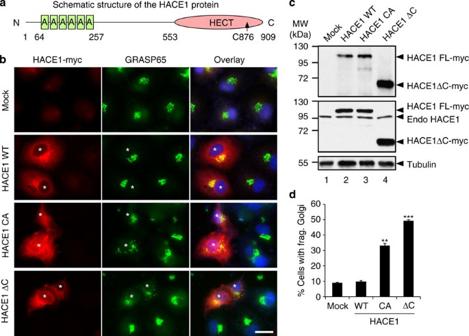Figure 5: Expression of HACE1 mutants leads to Golgi fragmentation. (a) Schematic structure of HACE1. It contains six ankyrin repeats at the N terminus and a HECT domain at the C terminus. Cysteine 876 has been shown to be essential for the ubiquitin ligase activity. A construct with the HECT domain deleted (ΔC, amino acids 1–553) was used in this study. (b) HeLa cells expressing myc-tagged WT HACE1 protein, the inactive C876A (CA) mutant and the ΔC mutant. Mock transfection with the empty vector. Asterisks indicate transfected cells. Note that expression of the CA and ΔC mutants leads to Golgi fragmentation. Scale bar, 20 μm. (c) Western blots illustrating that the correct proteins were expressed. Endo HACE1 refers to endogenous HACE1. (d) Quantification of Golgi fragmentation in 300 myc-tagged HACE1-expressing cells for each set of experiments. Shown are representative results (mean±s.e.m.) from three independent experiments. Statistical significance was assessed by comparison to the mock transfection.P-value was determined by Student'st-test; **P<0.005; ***P<0.001. Figure 5: Expression of HACE1 mutants leads to Golgi fragmentation. ( a ) Schematic structure of HACE1. It contains six ankyrin repeats at the N terminus and a HECT domain at the C terminus. Cysteine 876 has been shown to be essential for the ubiquitin ligase activity. A construct with the HECT domain deleted (ΔC, amino acids 1–553) was used in this study. ( b ) HeLa cells expressing myc-tagged WT HACE1 protein, the inactive C876A (CA) mutant and the ΔC mutant. Mock transfection with the empty vector. Asterisks indicate transfected cells. Note that expression of the CA and ΔC mutants leads to Golgi fragmentation. Scale bar, 20 μm. ( c ) Western blots illustrating that the correct proteins were expressed. Endo HACE1 refers to endogenous HACE1. ( d ) Quantification of Golgi fragmentation in 300 myc-tagged HACE1-expressing cells for each set of experiments. Shown are representative results (mean±s.e.m.) from three independent experiments. Statistical significance was assessed by comparison to the mock transfection. P -value was determined by Student's t -test; ** P <0.005; *** P <0.001. Full size image Previous experiments have suggested that ubiquitin has a role in p97/p47-mediated postmitotic Golgi membrane fusion [20] , [21] , it is possible that HACE1 functions in the same ubiquitination–deubiquitination pathway. Therefore, we used the standard Golgi disassembly and reassembly assay [7] to test the role of HACE1 in regulation of Golgi membrane dynamics. We first treated purified Golgi membranes with mitotic cytosol (MC) to induce membrane fragmentation. These mitotic Golgi fragments were further treated with interphase cytosol. After incubation, membranes were examined by electron microscopy (EM) and the percentage of membranes in cisternae was quantified [21] , [28] . To manipulate HACE1 activity, we added affinity-purified anti-HACE1 antibodies, or purified WT HACE1 or C876A mutant proteins into either the disassembly or the reassembly reactions. 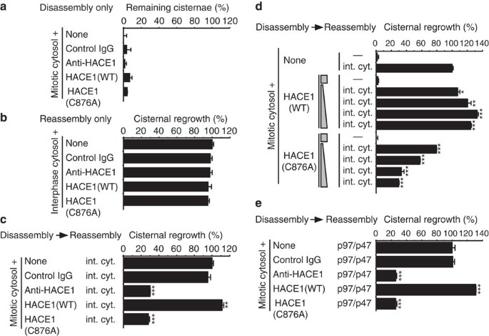Figure 6: HACE1 regulates p97/p47-mediated postmitotic Golgi membrane reassemblyin vitro. (a,b) HACE1 in mitotic Golgi disassembly or postmitotic reassembly. Purified rat Golgi was treated with mitotic cytosol (mit. cyt.), then with interphase cytosol. Control rabbit IgG, affinity-purified anti-HACE1 antibodies or purified proteins of WT HACE1 or the C876A mutant were added into the disassembly (a) or reassembly (b) reactions, as indicated. Membranes were processed for EM, and the results were quantified to estimate the percentage of cisternal membranes. Mitotic Golgi fragments (none, 23.6±1.1% membranes in cisternae) were normalized to 0%. Reassembly in interphase cytosol without any additional components (none, 57.1±0.5% membranes in cisternae) was normalized to 100%. (c) HACE1 ubiquitin ligase activity in mitotic Golgi disassembly is required for subsequent postmitotic Golgi membrane reassembly. Golgi membranes were fragmented by mitotic cytosol in the presence of the indicated reagents and incubated with interphase cytosol (int. cyt.). (d) HACE1 ligase activity levels correlate with the efficiency of postmitotic Golgi membrane assembly in a dose-dependent manner. Same as in (c), except with a serial increasing amount (0.1–1 μM) of purified WT HACE1 or C876A mutant included in the reassembly reactions. 0% represents mitotic Golgi fragments treated with mitotic cytosol and then fixed (24.1±0.6% membranes in cisternae), and 100% represents membranes reassembled in interphase cytosol (58.5±0.5% membranes in cisternae). (e) HACE1 affects p97/p47-mediated membrane fusion. Same as in (c), except that mitotic Golgi membranes were subsequently incubated with the purified p97/p47 proteins instead of interphase cytosol. 0% represents mitotic Golgi fragments treated with mitotic cytosol and then fixed (26.5±0.1% membranes in cisternae), and 100% represents membranes reassembled with p97/47 (53.6±1.1% membranes in cisternae). The results represent the mean of three independent experiments±s.e.m.P-value was determined by Student'st-test; *P<0.05; **P<0.005; ***P<0.001. As shown in Figure 6 , manipulation of HACE1 activity in the Golgi membrane disassembly reaction alone ( Fig. 6a ) or in the reassembly alone ( Fig. 6b ) had no effect. Figure 6: HACE1 regulates p97/p47-mediated postmitotic Golgi membrane reassembly in vitro . ( a , b ) HACE1 in mitotic Golgi disassembly or postmitotic reassembly. Purified rat Golgi was treated with mitotic cytosol (mit. cyt. ), then with interphase cytosol. Control rabbit IgG, affinity-purified anti-HACE1 antibodies or purified proteins of WT HACE1 or the C876A mutant were added into the disassembly ( a ) or reassembly ( b ) reactions, as indicated. Membranes were processed for EM, and the results were quantified to estimate the percentage of cisternal membranes. Mitotic Golgi fragments (none, 23.6±1.1% membranes in cisternae) were normalized to 0%. Reassembly in interphase cytosol without any additional components (none, 57.1±0.5% membranes in cisternae) was normalized to 100%. ( c ) HACE1 ubiquitin ligase activity in mitotic Golgi disassembly is required for subsequent postmitotic Golgi membrane reassembly. Golgi membranes were fragmented by mitotic cytosol in the presence of the indicated reagents and incubated with interphase cytosol (int. cyt.). ( d ) HACE1 ligase activity levels correlate with the efficiency of postmitotic Golgi membrane assembly in a dose-dependent manner. Same as in ( c ), except with a serial increasing amount (0.1–1 μM) of purified WT HACE1 or C876A mutant included in the reassembly reactions. 0% represents mitotic Golgi fragments treated with mitotic cytosol and then fixed (24.1±0.6% membranes in cisternae), and 100% represents membranes reassembled in interphase cytosol (58.5±0.5% membranes in cisternae). ( e ) HACE1 affects p97/p47-mediated membrane fusion. Same as in ( c ), except that mitotic Golgi membranes were subsequently incubated with the purified p97/p47 proteins instead of interphase cytosol. 0% represents mitotic Golgi fragments treated with mitotic cytosol and then fixed (26.5±0.1% membranes in cisternae), and 100% represents membranes reassembled with p97/47 (53.6±1.1% membranes in cisternae). The results represent the mean of three independent experiments±s.e.m. P -value was determined by Student's t -test; * P <0.05; ** P <0.005; *** P <0.001. Full size image Our previous results have demonstrated that ubiquitination occurs during Golgi disassembly and is required for subsequent reassembly [21] ; therefore, HACE1 may function in disassembly, which impacts subsequent Golgi reassembly. To test this idea, we first treated purified Golgi membranes with MC in the presence of either HACE1 recombinant protein or HACE1 antibodies and used the resulting Golgi fragments for reassembly. The addition of anti-HACE1 antibodies or the inactive HACE1 C876A mutant protein inhibited subsequent Golgi membrane reassembly. In contrast, the addition of WT HACE1 protein enhanced the subsequent Golgi membrane reassembly ( Fig. 6c ). These results suggest that the HACE1 ubiquitin ligase activity in mitotic Golgi membrane disassembly is required for subsequent postmitotic Golgi membrane reassembly. To ensure that the observed effects resulted from the addition of HACE1, we titrated different amounts of HACE1 recombinant protein into the disassembly reaction and used the membranes for subsequent reassembly. Higher concentrations of the WT HACE1 protein increased the stimulatory effects, whereas increasing the amount of HACE1 C876A mutant aggravated the inhibitory effects ( Fig. 6d ). These results show that HACE1 ligase activity levels are correlated with the efficiency of postmitotic Golgi membrane assembly in a dose-dependent manner. We then used the defined Golgi disassembly and reassembly assay [7] to determine whether HACE1 functions through p97/p47-mediated membrane fusion. Similar to the experiments described above, HACE1 antibodies and purified proteins were added to the disassembly reactions, and the generated mitotic Golgi membranes were subsequently incubated with purified p97/p47 proteins. As shown in Fig. 6e , the addition of anti-HACE1 antibodies or the purified HACE1 C876A mutant protein inhibited Golgi membrane reassembly, in contrast with the stimulatory effect of the WT protein. As the experimental conditions were optimized for Golgi membrane fusion, the increased reassembly efficiency caused by the addition of WT HACE1 strengthened the conclusion that HACE1 is involved in the regulation of Golgi membrane dynamics. Taken together, these results strongly suggest that HACE1 ubiquitin ligase activity in mitotic Golgi disassembly is required for p97/p47-mediated postmitotic Golgi membrane reassembly in vitro . HACE1 regulates Golgi membrane fusion in cells To determine whether HACE1 is needed for Golgi integrity in vivo , we reduced cellular HACE1 level using small interfering RNAs (siRNA; Fig. 7a,b ). Four pairs of RNA oligos were tested, and the most efficient pair was selected. HACE1 mRNA levels determined by real-time PCR (RT–PCR) were reduced by 66.8±4.8 and 74.1±4.3%, 2 and 4 days after transfection, respectively. At the protein level, there was a 62.0±4.8% reduction 4 days after transfection ( Fig. 7c ).These results indicate that endogenous HACE1 is a relatively stable protein. Indeed, when cells were treated with the protein synthesis inhibitor cycloheximide for 24 h, HACE1 protein levels were not significantly affected; in contrast, the same treatment caused a noticeable reduction of GRASP65 ( Supplementary Fig. S3a ). To confirm the specificity of our siRNA oligos, HeLa cells were transiently transfected with a HACE1-myc cDNA and HACE1 or control siRNA oligos. HACE1-myc was expressed well when cotransfected with the control siRNA but not with the HACE1 siRNA ( Supplementary Fig. S3b ). These results confirmed that the siRNA used to deplete the HACE1 mRNA and protein is specific and, to some degree, effective. 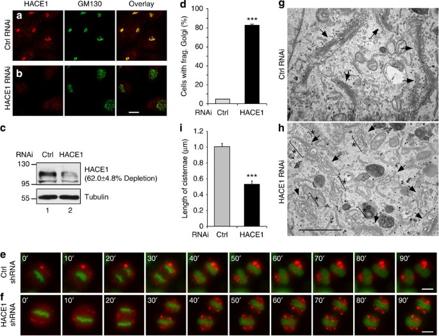Figure 7: Depletion of HACE1 leads to Golgi fragmentation. (a,b) Confocal fluorescence images of HACE1 knockdown cells. HeLa cells transfected with the indicated siRNA oligos were fixed and stained for HACE1 and GM130. Scale bars in all panels, 20 μm. (c) Immunoblots of HeLa cells described ina,b. The knockdown efficiency of HACE1 protein was 62.0±4.8% from three independent experiments. (d) Quantification of the fluorescence images in (a,b) from three independent experiments. Shown is the percentage of cells with fragmented Golgi (frag. golgi), and 300 cells were counted for each experiment. The results expressed are the means±s.e.m. (e,f) HACE1 depletion delays postmitotic Golgi formation. HeLa cells were infected by control lentivirus (e) or lentivirus that expresses HACE1 shRNA (f). Cells were then cotransfected with cDNAs for Histone H2B–GFP (in green) and α-mannosidase II–mCherry (in red) followed by time-lapse microscopy in 10 min intervals over 3 h (seeSupplementary Movies 1-2). The frame of metaphase cells with aligned chromosomes right before chromosome separation (the onset of anaphase) were set to 0 time point. Scale bar, 10 μm. (g,h) Representative EM micrographs of the cells described in (a,b). The arrowheads indicate Golgi stacks, and asterisks indicate fragmented cisternal membranes. Scale bar, 1 μm. Note that the Golgi ribbon in HACE1-depleted cells is disorganized, and the cisternae are shorter compared with control siRNA-treated cells. (i) Quantification of the EM images in (g,h) from three independent experiments. Note that cisternal length is reduced by HACE1 depletion. Statistical significance was assessed by comparison to the control siRNA-treated cells.P-value was determined by Student'st-test; ***P<0.001. Figure 7: Depletion of HACE1 leads to Golgi fragmentation. ( a , b ) Confocal fluorescence images of HACE1 knockdown cells. HeLa cells transfected with the indicated siRNA oligos were fixed and stained for HACE1 and GM130. Scale bars in all panels, 20 μm. ( c ) Immunoblots of HeLa cells described in a , b . The knockdown efficiency of HACE1 protein was 62.0±4.8% from three independent experiments. ( d ) Quantification of the fluorescence images in ( a , b ) from three independent experiments. Shown is the percentage of cells with fragmented Golgi (frag. golgi), and 300 cells were counted for each experiment. The results expressed are the means±s.e.m. ( e , f ) HACE1 depletion delays postmitotic Golgi formation. HeLa cells were infected by control lentivirus ( e ) or lentivirus that expresses HACE1 shRNA ( f ). Cells were then cotransfected with cDNAs for Histone H2B–GFP (in green) and α-mannosidase II–mCherry (in red) followed by time-lapse microscopy in 10 min intervals over 3 h (see Supplementary Movies 1-2 ). The frame of metaphase cells with aligned chromosomes right before chromosome separation (the onset of anaphase) were set to 0 time point. Scale bar, 10 μm. ( g , h ) Representative EM micrographs of the cells described in ( a , b ). The arrowheads indicate Golgi stacks, and asterisks indicate fragmented cisternal membranes. Scale bar, 1 μm. Note that the Golgi ribbon in HACE1-depleted cells is disorganized, and the cisternae are shorter compared with control siRNA-treated cells. ( i ) Quantification of the EM images in ( g , h ) from three independent experiments. Note that cisternal length is reduced by HACE1 depletion. Statistical significance was assessed by comparison to the control siRNA-treated cells. P -value was determined by Student's t -test; *** P <0.001. Full size image We then analysed the Golgi morphology in HACE1-depleted cells. These cells had reduced signal for HACE1 when analysed by fluorescence microscopy ( Fig. 7a,b ). Depletion of HACE1 led to Golgi fragmentation using GM130 ( Fig. 7b versus Fig. 7a ), GRASP65 or syntaxin 5 (data not shown) as Golgi markers; 83.0±0.9% of the HACE1-depleted cells exhibited Golgi fragmentation, a significant increase compared with control siRNA transfected cells (4.8±0.2%, Fig. 7d ). As in vitro experiments indicate that HACE1 is involved in postmitotic Golgi reassembly, we monitored the reformation of Golgi ribbon in control or HACE1-depleted cells using time-lapse microscopy. We infected HeLa cells by lentivirus packaged either an empty vector or a vector-encoding HACE1 short-hairpin RNA (shRNA) and generated stable cells. The knockdown efficiency of the HACE1 protein in these cells was similar to HACE1 siRNA transfection, as assessed by western blot ( Supplementary Fig. S3 ). Control cells or HACE1 shRNA-expressing cells were then cotransfected with cDNAs encoding α-mannosidase II–mCherry to label the Golgi membranes and Histone H2B–GFP to visualize the morphology of the chromosomes in the cells. Metaphase cells with aligned chromosomes were then analysed by time-lapse microscopy for postmitotic Golgi formation. The frame right before chromosome separation (the onset of anaphase) was set to 0 time point. Golgi reassembly was completed within 80±5 min in control siRNA-treated cells; while in HACE1 knockdown cells, the Golgi remained fragmented 180 min after the onset of anaphase ( Fig. 7e,f ; Supplementary Movies 1-2 ). These results demonstrate that HACE1 depletion impairs postmitotic Golgi reassembly. We then examined the Golgi structure more closely by EM. Control siRNA-transfected cells showed well-organized stacks, which often aligned in parallel to form a ribbon. In contrast, HACE1-depleted cells had fragmented Golgi. The Golgi membranes were disorganized and the cisternae were relatively short, while a large part of the membranes were vesiculated, and small stacks or single cisterna were dispersed throughout the cells and did not form a ribbon ( Fig. 7h versus g ). The average cisternal length was reduced from 1.01±0.04 μm in control siRNA-transfected cells to 0.53±0.04 μm in HACE1-depleted cells ( Fig. 7i ). These results suggest that HACE1 depletion reduces membrane fusion activity, which may subsequently impair Golgi ribbon linking observed as fragmented Golgi under the light microscope ( Figs 5b,d and 7b,d,f ). It has been previously observed that the SK-NEP-1 cell line expresses relatively low level of HACE1 protein [26] ; therefore, we examined the Golgi morphology in these cells in comparison with HeLa cells ( Fig. 8a,b ). Indeed, HACE1 protein level in this cell line was 30.9±3.1% compared with HeLa cells as determined by western blots ( Fig. 8c ). The expression levels of HACE1 were similar in several cell lines, such as HeLa, A431 and NRK cells (data not shown). When analysed by fluorescence microscopy, a large number of SK-NEP-1 cells showed fragmented Golgi. Compared with HeLa cells ( Fig. 8b ) and several other cell lines in which the Golgi membranes were well organized into a perinuclear ribbon-like structure, the Golgi membranes in SK-NEP-1 cells were disconnected, not localized to the perinuclear region and dispersed throughout the cell. Fragmented Golgi structures were observed in 34.9±2.2% of the SK-NEP-1 cells compared with 5.6±1.0% in HeLa cells ( Fig. 8a,d ), suggesting that these cells had a possible Golgi membrane fusion defect. 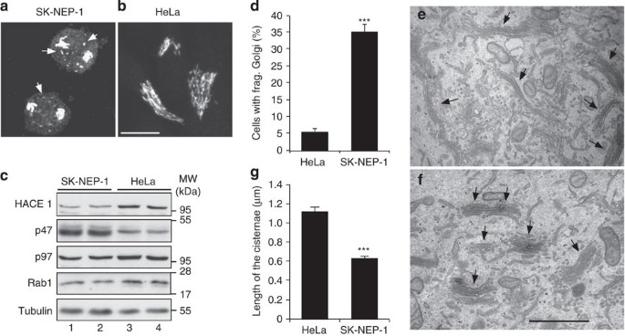Figure 8: The Golgi apparatus is fragmented in SK-NEP-1 cells that have reduced HACE1 expression. (a,b) Representative fluorescence images of SK-NEP-1 cells showing that the Golgi indicated by GRASP65 is fragmented compared with HeLa cells. Arrows indicate isolated Golgi fragments. Scale bar, 10 μm. (c) HACE1 expression is reduced in SK-NEP-1 cells. Western blot detecting HACE1, tubulin, p97 and p47 in HeLa cells and SK-NEP-1 cell lysates. (d) Quantification of the number of HeLa and SK-NEP-1 cells containing fragmented Golgi. (e,f) EM images of (e) HeLa and (f) SK-NEP-1 cells. Scale bar, 1 μm. Note that SK-NEP-1 cells have isolated stacks with relatively short cisternae. (g) Quantification of the EM images in (e,f) from three independent experiments. The average length of the cisternae in HeLa cells was 1.12±0.05 μm (mean±s.e.m.), while in SK-NEP-1 cells it was 0.63±0.02 μm.P-value was determined by Student'st-test; ***P<0.001. Figure 8: The Golgi apparatus is fragmented in SK-NEP-1 cells that have reduced HACE1 expression. ( a , b ) Representative fluorescence images of SK-NEP-1 cells showing that the Golgi indicated by GRASP65 is fragmented compared with HeLa cells. Arrows indicate isolated Golgi fragments. Scale bar, 10 μm. ( c ) HACE1 expression is reduced in SK-NEP-1 cells. Western blot detecting HACE1, tubulin, p97 and p47 in HeLa cells and SK-NEP-1 cell lysates. ( d ) Quantification of the number of HeLa and SK-NEP-1 cells containing fragmented Golgi. ( e , f ) EM images of ( e ) HeLa and ( f ) SK-NEP-1 cells. Scale bar, 1 μm. Note that SK-NEP-1 cells have isolated stacks with relatively short cisternae. ( g ) Quantification of the EM images in ( e , f ) from three independent experiments. The average length of the cisternae in HeLa cells was 1.12±0.05 μm (mean±s.e.m. ), while in SK-NEP-1 cells it was 0.63±0.02 μm. P -value was determined by Student's t -test; *** P <0.001. Full size image The SK-NEP-1 cells were then analysed by EM in parallel with HeLa cells. HeLa cells contained well-organized stacks that often aligned into a ribbon-like structure ( Fig. 8e ), whereas in SK-NEP-1 cells the Golgi structure was less well organized. The cisternae were often not aligned into stacks, and the stacks were often more dispersed. More importantly, cisternae were shorter compared with those in HeLa cells. The average length of the SK-NEP-1 cisternae was 0.63±0.02 μm, a significant reduction compared with that (1.12±0.05 μm) found in HeLa cells ( Fig. 8g ). Cisternal length was similar in several cell lines tested, including HeLa, NRK and CHO cells (data not shown). These results agree with the HACE1 knockdown experiment, suggesting that HACE1 regulates Golgi membrane fusion. Taken together, these results demonstrate that HACE1 has a critical role in Golgi biogenesis during the cell cycle. We have identified the ubiquitin ligase HACE1 that interacts with Rab1 and is targeted to the Golgi membrane. Its activity in mitotic Golgi disassembly is required for subsequent postmitotic Golgi reassembly mediated by the p97/p47 complex. Depletion of HACE1, or expression of inactive HACE1 mutants, reduced the length of cisternae in the stacks and affected the overall Golgi structure. HACE1 depletion had stronger effect on the Golgi structure than the expression of inactive HACE1; this is likely due to three possible reasons. First, the mutants of HACE1 may not function as strong dominant negative mutants to inhibit the endogenous HACE1. Second, the effect of the exogenous protein may be concentration-dependent and the expression level in the cells is heterogeneous. Third, HACE1 exhibits its activity during mitotic Golgi disassembly, which is required for the subsequent Golgi reassembly. Therefore, the effect on the Golgi morphology may require one or more cycles of cell division. The cells transfected with siRNA were examined 96 h after transfection, whereas the cells expressing the mutant proteins were examined about 16 h after transfection. Most of the siRNA transfected cells should have gone through at least one cell cycle, whereas the percentage of mutant HACE1-expressing cells that went through mitosis was much lower. Nevertheless, these findings provided evidence that HACE1 is a key regulator of Golgi membrane dynamics during the cell cycle. The tight interaction between HACE1 and Rab1 also suggests that HACE1 is an effector of Rab1 GTPases. The expression of Rab1 inactive mutant caused dissociation of HACE1 from the Golgi membranes and Golgi fragmentation, suggesting that Rab1 has a critical role for HACE1 function on the Golgi membranes. This result is consistent with the requirement of a functional Rab1 for Golgi structure and function [37] . HACE1 was previously identified as a critical tumour suppressor involved in multiple cancers, such as sporadic Wilms' tumour [26] , [27] , [38] . The mechanism by which HACE1 depletion leads to cancer formation, however, remains elusive. One attractive hypothesis is that the role of HACE1 in cell proliferation is related to its role in regulating Golgi biogenesis during the cell cycle. The Golgi is the central machinery for protein modification, processing, trafficking and secretion. Defects in the Golgi structure and function may directly affect cell growth and proliferation. Golgi defects may also impair the accuracy of protein glycosylation, including cell adhesion molecules on cell surface, which may lead to metastasis. Indeed, abnormal Golgi division has been observed in cancer cells [39] , and defects in protein processing and secretion have been related to cancer cell metastasis [40] , [41] , [42] . The mechanism by which ubiquitination and deubiquitination regulate Golgi dynamics remains elusive. It has been shown that the activity of the VCIP135 deubiquitinating enzyme is required for postmitotic Golgi membrane fusion [21] . Therefore, it is likely that at least one Golgi membrane protein is ubiquitinated by HACE1 when the Golgi undergoes mitotic fragmentation. Monoubiquitination does not result in the degradation of the substrate; instead, it recruits the p97/p47 complex to the Golgi membrane through interaction between the p47 UBA domain and ubiquitin [20] , [21] . Subsequently, the p97/p47 complex recruits VCIP135 to the membrane. When the ubiquitin is removed from the substrate(s) by VCIP135, the membranes are subjected to p97/p47-mediated fusion. Consistently, our in vivo and in vitro experiments demonstrate that the lack of HACE1 activity reduces Golgi membrane fusion and results in short cisternae, possibly because of the reduced recruitment of the p97/p47 complex to the membranes. The reduced cisternal length in the stacks resulted from HACE1 depletion also suggests that membrane fusion mediated by NSF, another machinery in postmitotic Golgi membrane fusion, cannot compensate the loss of p97 (and ubiquitin)-mediated membrane fusion activity. Consistent with this, it has been shown that NSF- and p97-mediated Golgi reassembly pathways contribute non-additively to cisternal regrowth [15] , but the coordination between two pathways has not been fully elucidated. Our results suggest a mechanism by which ubiquitination functions as a signal that regulates Golgi reassembly after cell division. The key question for understanding the mechanism requires the identification of the ubiquitinated substrate(s), which will help determine whether the lack of Golgi membrane fusion activity during mitosis is due to ubiquitination of Golgi membrane proteins. It is tempting to speculate that the target in this pathway is part of the membrane fusion machinery that includes SNAREs and SNARE-interacting proteins as well as the key Golgi structural proteins such as Golgins and GRASP proteins. Further experiments are necessary to identify these substrates on the Golgi membrane and to determine how HACE1 activity is regulated during the cell cycle. Reagents All reagents were purchased from Sigma-Aldrich, Roche or Calbiochem, unless otherwise stated. The following antibodies were used: monoclonal antibodies against ERGIC53 (Peter Arvan), Gos28 and GM130 (Transduction Laboratories), myc (Dr David Sheff), syntaxin 6 (BD Biosciences) and α-tubulin (Developmental Studies Hybridoma Bank University of Iowa); polyclonal antibodies against protein disulphide isomerase (Peter Arvan), GFP [11] , GM130 (ref. 8 ), rat GRASP55 (ref. 11 ), GRASP65 (ref. 10 ), α-mannosidase II (Dr Graham Warren), p47 and p97 (ref. 21 ), Rab1A, Rab6 and Rab11 (ref. 43 ) and sec61α (Upstate). The HACE1 antibody was generated in rabbits using recombinant GST–HACE1 (amino acids 1–548) as the immunogen and subsequently affinity purified; it was used at 1:1000 dilution for western blot and 1:100 for fluorescence microscopy. The GalNAc-T2-GFP cDNA was a gift from Dr Graham Warren. Secondary antibodies were from Jackson Lab and Invitrogen. The GST–Rab1a (WT, Q67L and S25N) and GST–Rab2 cDNA constructs were kindly provided by Dr Graham Warren. The GST–Rab5, GST–Rab6 and GST–Rab11 plasmids were a gift from Dr Suzanne Pfeffer. GFP-tagged Rab4 (WT, Q67L and S22N) constructs were from Dr Stephen Ferguson. GFP–Rab11 (WT, Q70L and S25N) constructs were from Dr David Sheff. HACE1 identification and Rab interaction To purify Rab4 effectors, GST–Rab4 was expressed in 20 l of DH5α cells and bound to 2 ml of glutathione beads (GE Healthcare). The sample was equally divided into two tubes and incubated with nucleotide-exchange buffer (20 mM Hepes-KOH, pH 7.5, 100 mM NaCl, 10 mM EDTA, 5 mM MgCl 2 and 1 mM dithiothreitol (DTT)), containing 1 mM GTPγS in one tube and 1 mM GDP in the other, for 20 min at room temperature with rotation. This step was repeated three times. GST–Rab4 bound to beads was then stabilized with nucleotide-stabilization buffer (NS buffer; 20 mM Hepes-KOH, pH 7.5, 100 mM NaCl, 5 mM MgCl 2 and 1 mM DTT) in the presence of 1 mM GTPγS or GDP for 20 min at room temperature with rotation. Beads were then incubated with 50 ml of bovine brain cytosol (20 mg ml −1 ) [25] for 2 h at 4 °C. After incubation, the beads were washed with ten column volumes of NS buffer with 10 μM GTPγS or GDP; 10 volumes of NS buffer containing 250 mM NaCl and 10 μM GTPγS or GDP and 1 volume of 20 mM Hepes-KOH, pH 7.5, 250 mM NaCl and 1 mM DTT. To elute the bound proteins, the beads were incubated with 1.5 column volumes of elution buffer (20 mM Hepes-KOH, pH 7.5, 1.5 M NaCl, 20 mM EDTA, 1 mM DTT and 5 mM GDP) for 20 min at room temperature with rotation. Eluted proteins were analysed by SDS–PAGE and coomassie blue staining. The bands in the GTPγS lane were excised and analysed by mass spectrometry. The generated peptide sequences were searched in the NCBI EST database. The full-length HACE1 cDNA clone was isolated by screening a SUPERSCRIPT HeLa cDNA library, which was subsequently cloned into the pGEX-6p-1 vector for bacterial expression and pCDNA3.1 for mammalian expression (see Supplementary Methods for further details). The interactions between HACE1 and Rab were determined by a pull-down assay following a previously established procedure [28] , with details described in the Supplementary Methods . Thioester bond formation assay To test whether HACE1 is an active ubiquitin ligase, 60 nM recombinant human ubiquitin activating enzyme E1 (Biomol International), 200 nM recombinant human UbcH7 (Biomol International) [26] , 19 μM biotinylated ubiquitin and 600 nM recombinant GST-tagged WT or mutant HACE1 were mixed in 40 μl reactions in reaction buffer that contained 20 mM Tris–HCl, pH 7.4,. 50 mM KCl, 5 mM MgCl 2 , 2 mM ATP, 0.2 M sucrose and protease inhibitors (Roche). Reactions were incubated at 30 °C for 60 min and mixed with SDS–PAGE sample buffer with or without DTT followed by detection of HACE1 by western blot. Cell culture and microscopy HeLa and NRK cells were routinely cultured in Dulbecco's Modified Eagle Medium supplemented with 7.5% fetal calf serum, 2 mM L -glutamine, penicillin (100 U ml −1 ) and streptomycin (100 μg ml −1 ). SK-NEP-1 cells were cultured in McCoy's medium with 15% fetal calf serum. For nocodazole treatment, cells were treated with 0.5 μg ml −1 nocodazole for 2 h followed by fluorescence microscopy. For BFA treatment and washout, cells were treated with 5 μg ml −1 BFA for 2 h, washed twice with PBS and further incubated in growth media for 2 h. siRNA oligos were designed using the Invitrogen BLOCK-iT RNAi Designer software according to the human HACE1 sequence (sense: 5′-UAUAGCGCUGAUGUCAACA(TT)-3′, antisense: 5′-UGUUGACAUCAGCGCUAUA(TT)-3′). In a previous report [27] , three pairs of RNA oligos from Invitrogen were used to deplete HACE1. These oligos were less effective at knocking down HACE1 than our newly designed oligos. HeLa and HEK 293T cells were transfected using Lipofectamine RNAiMAX (Invitrogen) following the manufacturer's instructions. Control transfections were performed simultaneously using non-specific siRNA oligos purchased from Ambion. Assays were performed 96 h after transfection unless otherwise stated. Depletion efficiency of endogenous HACE1 was quantified from the western blot results using the NIH ImageJ software and normalized to tubulin levels. To construct HACE1 knockdown stable cell lines, HeLa cells were infected by MISSION HACE1 shRNA lentiviral particles (Sigma, product # SHCLNV-NM_020771, contains five shRNA lentiviral clones) and transduced cells were selected by the addition of 1 μg ml −1 puromycin into the culture medium. Among the five HACE1 shRNA lentiviral clones, clone TRCN0000003414 gave the best knockdown efficiency examined by western blots ( Supplementary Fig. S3 ). Lentivirus packaged with the pLentilox3.7-GFP vector was obtained from the University of Michigan Vector Core and used as a control. For expression of exogenous HACE1, HeLa cells were transfected with the indicated HACE1 constructs using Lipofectamine 2000 (Invitrogen). Methods for subcellular fractionation, microscopy and statistical analysis are described in Supplementary Methods . RT–PCR mRNA was purified from a 6-cm dish of HeLa cells using RNeasy columns (QIAGEN Inc.). First-strand cDNA was synthesized using Superscript III RT (Invitrogen) and utilized for semiquantitative RT–PCR using IQ SYBR Green Supermix (Bio-Rad). A Bio-Rad IQ iCycler was used to measure the expression levels of transcripts. The HACE1 mRNA level was normalized to glyceraldehyde 3-phosphate dehydrogenase. Intron-spanning primers are designed using the 'Primer 3' software. The following primer sequences were used for HACE1: forward primer: 5′-GCTCTTGCAGGGAGACAGGA-3′, reverse primer: 5′-AGTCATTCCCGGAGGCATCT-3′. The glyceraldehyde 3-phosphate dehydrogenase primers were provided by Dr Haoxing Xu [44] . Forward primer: 5′-GAAGGTGAAGGTCGGAGTCA-3′, reverse primer: 5′-AATGAAGGGGTCATTGATGG-3′. Golgi disassembly and reassembly assay, and quantification Golgi membranes were purified from rat liver [45] . Interphase cytosol (IC) and MC were prepared from HeLa S3 cells [5] . His-tagged p47 was expressed in bacteria and purified using nickel beads [20] . p97 was prepared using a bacterial expression system or purified from rat liver cytosol by gel filtration [17] , [20] . The Golgi disassembly assay was performed as described previously [6] . Briefly, purified Golgi membranes (20 μg) were mixed with 2 mg of mitotic cytosol, 1 mM GTP and an ATP-regenerating system (10 mM creatine phosphate, 1 mM ATP, 20 μg ml −1 creatine kinase and 20 ng ml −1 cytochalasin B) in MEB buffer (50 mM Tris–HCl, pH 7.4, 0.2 M sucrose, 50 mM KCl, 20 mM β-glycerophosphate, 15 mM EGTA, 10 mM MgCl 2 , 2 mM ATP, 1 mM GTP, 1 mM glutathione and protease inhibitors) in a final volume of 200 μl. In some reactions, 1 μM or an increasing amount (0.1–1 μM) of WT or mutant HACE1 recombinant proteins or 10 ng μl −1 anti-HACE1 antibodies were added into the disassembly assay as indicated. After incubation for 60 min at 37 °C, mitotic Golgi fragments were isolated and soluble proteins were removed by centrifugation (135,000 g for 30 min in a TLA55 rotor) through a 0.4-M sucrose cushion in KHM buffer (20 mM Hepes-KOH, pH 7.0, 0.2 M sucrose, 60 mM KCl, 5 mM Mg(OAc) 2 , 2 mM ATP, 1 mM GTP, 1 mM glutathione and protease inhibitors) onto a 6-μl 2 M sucrose cushion. The membranes were resuspended in KHM buffer and were either fixed and processed for EM [6] , [10] , [12] or used in reassembly reactions. For Golgi reassembly, 20 μg of Golgi fragments were resuspended in KHM buffer, mixed with either 400 μg IC or 100 ng μl −1 p97 and 25 ng μl −1 p47 in KHM buffer in the presence of an ATP regeneration system in a final volume of 30 μl and incubated at 37 °C for 60 min. The membranes were pelleted by centrifugation, and processed for EM. For EM analysis, the percentage of membranes in cisternae or in vesicles was determined by the intersection method [4] , [10] . Cisternae were defined as long membrane profiles with a length greater than four times their width, and the latter did not exceed 60 nm. Normal cisternae ranged from 20 to 30 nm in width and were longer than 200 nm. Stacks were defined as two or more cisternae that were separated by no more than 15 nm and overlapped in parallel by more than 50% of their length. All experiments were repeated at least three times; statistical significance was assessed by Student's t -test. See Supplementary Methods for further details on HACE1 cloning, expression, Rab interaction, subcellular localization and microscopy. How to cite this article: Tang, D. et al . The ubiquitin ligase HACE1 regulates Golgi membrane dynamics during the cell cycle. Nat. Commun. 2:501 doi: 10.1038/ncomms1509 (2011).